Experimental evolution of an alternating uni- and multicellular life cycle inChlamydomonas reinhardtii The transition to multicellularity enabled the evolution of large, complex organisms, but early steps in this transition remain poorly understood. Here we show that multicellular complexity, including development from a single cell, can evolve rapidly in a unicellular organism that has never had a multicellular ancestor. We subject the alga Chlamydomonas reinhardtii to conditions that favour multicellularity, resulting in the evolution of a multicellular life cycle in which clusters reproduce via motile unicellular propagules. While a single-cell genetic bottleneck during ontogeny is widely regarded as an adaptation to limit among-cell conflict, its appearance very early in this transition suggests that it did not evolve for this purpose. Instead, we find that unicellular propagules are adaptive even in the absence of intercellular conflict, maximizing cluster-level fecundity. These results demonstrate that the unicellular bottleneck, a trait essential for evolving multicellular complexity, can arise rapidly via co-option of the ancestral unicellular form. The transition to multicellularity was one of a few major events in life’s history that created new opportunities for more complex biological systems to evolve [1] . As this transition fundamentally changes what constitutes an individual, dissecting the steps in this transition remains a major challenge within evolutionary biology [2] . Compared with other major transitions in evolution that occurred just once (for example, the origin of eukaryotes [3] ), multicellularity has evolved repeatedly. Indeed, cyanobacteria evolved simple filamentous multicellularity over 2.5 billion years ago [4] , and entire clades of multicellular organisms have arisen in the last 200 million years (for example, brown algae [5] and the volvocine algae [6] ). Most origins of multicellularity are ancient and transitional forms have been lost to extinction [7] , so little is known about the potential for multicellularity to evolve from unicellular lineages, or the route through which a multicellular life history arises. Here we use experimental evolution [8] , [9] to directly examine the first steps in this transition using the unicellular alga Chlamydomonas reinhardtii . This species is uniquely suited to such an investigation, as it has never had a multicellular ancestor and is closely related to the volvocine algae, a clade in which the historical order of multicellular adaptations has been inferred [10] . Even within this lineage, there is evidence that multicellular forms with different levels of organization have evolved independently [10] . A hallmark feature of complex multicellularity is a two-stage life cycle in which multicellular individuals develop from a single cell [11] , [12] , [13] . While this process is often coupled with sexual reproduction, mitotically produced unicellular propagules are also widespread (for example, in multicellular red, green, and brown algae [14] and parthenogenetic animals [15] ). The ubiquity and persistence of the unicellular bottleneck has been attributed to the fact that it purges within-group genetic variation, eliminating the potential for among-cell evolutionary conflicts that might otherwise erode multicellular complexity [1] , [12] , [16] , [17] , [18] , [19] , [20] , [21] . Although there is little doubt that a unicellular bottleneck serves the present function of preventing among-cell conflicts in large multicellular organisms, there is no direct evidence that it originally arose as an adaptation for this function. This hypothesis is especially problematic for early (presumably small), clonally developing multicellular taxa where within-organism genetic variation is negligible and the potential for genetic conflict minimal. Instead, the unicellular bottleneck may have evolved in the absence of genetic conflict for other reasons, creating a multicellular body plan largely immune to future intercellular conflicts as a side-effect. This key trait may therefore catalyse the evolution of multicellular complexity, facilitating the origin and expansion of cellular division of labour. Here we report on the de novo evolution of a two-stage life cycle in the unicellular alga C. reinhardtii. Twenty replicate populations of outbred C. reinhardtii were grown unshaken in 24-well plates. Subsamples of these populations were transferred to fresh medium every 3 days for a total of 73 transfers (~315 generations). To select for cluster formation, the first step in the transition to multicellularity [22] , 10 populations were subjected to strong selection for rapid settling through liquid medium. Briefly, we performed the selection by centrifuging 1 ml of each population at 100 g for 5 s and then transferring only the bottom 100 μl to fresh medium. Ten control populations were transferred without settling selection. Like other selection regimes that favour increased size (for example, grazing by phagotrophic predators [23] ), settling selection favors larger clusters that settle rapidly [24] . Settling selection was used in place of predation because it provides several key experimental advantages. First, settling is more replicable than predation because it is simpler (for example, no potential for predator co-evolution, density-dependent size selection, extinction of predators, and so on). Second, the strength of selection can easily be modified by changing the intensity or duration of centrifugation. In our experiments, we find that simple multicellularity can evolve rapidly in C. reinhardtii . Like most extant multicellular organisms, we find that multicellular C. reinhardtii possesses a life history that alternates between uni- and multicellular stages. The unicellular genetic bottleneck is present very early in this transition, and a simple life history model shows that it provides a fitness benefit even in the absence of among-cell conflict. Given the unicellular ancestry of all multicellular organisms, the evolution of a single-cell genetic bottleneck by co-option of the ancestral phenotype may represent a rapid and general route by which this trait can arise. Response to selection Chlamydomonas rapidly evolved multicelled clusters in response to settling selection ( Fig. 1 ). A single selected population began to settle more quickly than the other 19 populations after 46 transfers; by 73 transfers the difference in settling speed was readily apparent ( Fig. 1a ). At this time point, only this single population had evolved to form multicellular clusters. Multicellular C. reinhardtii clusters are held together by a transparent extracellular matrix ( Fig. 1b ) and can contain hundreds of cells. Using time-lapse microscopy, we tracked the growth of a small cluster in liquid medium for 24 h. Significantly, clusters develop clonally by daughter cells ‘staying together’ after mitotic reproduction [25] ( Fig. 1e ), not by aggregation of single cells that cohabit the same growth chamber. 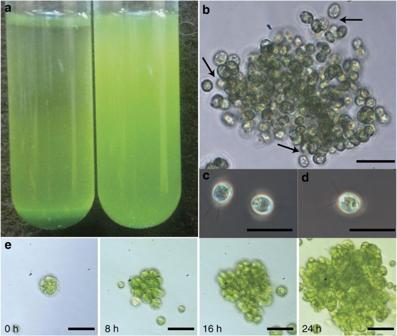Figure 1: MulticellularChlamydomonasmorphology. (a) MulticellularC. reinhardtii(left) settle faster than a contemporary population undergoing settling selection that remained unicellular (right), forming a pellet after 20 min of settling on the bench (cultures shown are 72 h old). (b) Cells are held in place by a transparent extracellular matrix, indicated by arrows. (c) Motile propagules released from multicellular clusters (phase contrast microscopy); (d) the ancestral unicellular growth form. Note thatcanddare phenotypically identical. (e) Cluster formation from a single cell. Cells form clusters by ‘staying together’ after mitotic reproduction, not aggregation of unrelated cells. All scale bars are 25 μm. Figure 1: Multicellular Chlamydomonas morphology. ( a ) Multicellular C. reinhardtii (left) settle faster than a contemporary population undergoing settling selection that remained unicellular (right), forming a pellet after 20 min of settling on the bench (cultures shown are 72 h old). ( b ) Cells are held in place by a transparent extracellular matrix, indicated by arrows. ( c ) Motile propagules released from multicellular clusters (phase contrast microscopy); ( d ) the ancestral unicellular growth form. Note that c and d are phenotypically identical. ( e ) Cluster formation from a single cell. Cells form clusters by ‘staying together’ after mitotic reproduction, not aggregation of unrelated cells. All scale bars are 25 μm. Full size image Life cycle To gain further insight into this multicellular life cycle, we analysed the growth of 10 isogenic isolates of multicellular C. reinhardtii from the 73-transfer population over a 72 h culture cycle. These isolates share complete sequence identity at five unlinked loci ( Table 1 ), suggesting they share a recent common ancestor. During the first 24 h of culture, actively swimming solitary cells ( Fig. 1c ) were present in the population ( Fig. 2a ), suggesting that clusters reproduce via motile unicells. To confirm this, we examined cluster-level reproduction using time-lapse microscopy. No cells dispersed from the cluster during the first four hours after transfer to fresh medium. After 4.16 h, cells in clusters began to activate their flagella, causing the cluster to convulse rapidly ( Fig. 2b ; Supplementary Movie 1 ). This change in state, from stasis to full movement, took 3 minutes ( Fig. 2b ). Six minutes after the onset of flagellar activity, the first motile individual cells broke free from the cluster. Five hours after transfer to fresh medium, many of the cells in the cluster had dispersed ( Supplementary Movie 1 ), which coincides with peak swimming activity observed at the population level ( Fig. 2a ). Clusters did not increase in size significantly during the first 24 h of culture ( Fig. 2c ; F 8,24 =26.8, ANOVA. P =0.98, assessed with Tukey–Kramer HSD). Table 1 Primers used in this study. 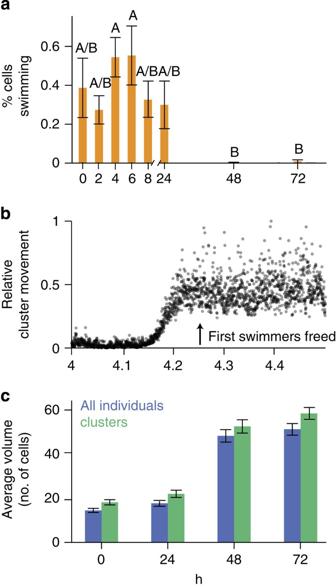Figure 2: MulticellularChlamydomonasalternate between motile unicells and sessile clusters. (a)C. reinhardtiiwere evolved by serial transfer every 72 h. Swimming unicells are abundant during the first 24 h of culture, but are virtually absent during the latter 48 h of the culture cycle. Time points demarcated by different letters (A, B) are significantly different at theα=0.05 level (F7,79=4.1, ANOVA;P=0.0008; differences between time points assessed with Tukey–Kramer HSD). Values shown in (a) are the mean±s.e.m. of 9 replicates per time point. (b) Flagella become active shortly after transfer to fresh medium, causing the cluster to convulse rapidly. Cluster movement was measured (relative to maximum displacement) using time-lapse microscopy. Maximum cluster movement was obtained after 4.25 hours, when the first motile unicellular propagules were released from the cluster. (c) Mean size of multicellularC. reinhardtiiincreased throughout the culture cycle. Cluster size remained constant during the dispersal phase (0–24 h), but increased nearly threefold during the growth phase (24–72 h). Error bars are the s.e.m. of 9 replicates per time point. Full size table Figure 2: Multicellular Chlamydomonas alternate between motile unicells and sessile clusters. ( a ) C. reinhardtii were evolved by serial transfer every 72 h. Swimming unicells are abundant during the first 24 h of culture, but are virtually absent during the latter 48 h of the culture cycle. Time points demarcated by different letters (A, B) are significantly different at the α =0.05 level ( F 7,79 =4.1, ANOVA; P =0.0008; differences between time points assessed with Tukey–Kramer HSD). Values shown in ( a ) are the mean±s.e.m. of 9 replicates per time point. ( b ) Flagella become active shortly after transfer to fresh medium, causing the cluster to convulse rapidly. Cluster movement was measured (relative to maximum displacement) using time-lapse microscopy. Maximum cluster movement was obtained after 4.25 hours, when the first motile unicellular propagules were released from the cluster. ( c ) Mean size of multicellular C. reinhardtii increased throughout the culture cycle. Cluster size remained constant during the dispersal phase (0–24 h), but increased nearly threefold during the growth phase (24–72 h). Error bars are the s.e.m. of 9 replicates per time point. Full size image During the last 48 h of the culture cycle, multicellular C. reinhardtii increased in volume by an average of 2.9-fold ( Fig. 2c , F 8,24 =31.6, ANOVA. p =0.013, Tukey–Kramer HSD). This size increase was due to cellular division within existing clusters, which grew an average of 2.7-fold during this time ( Fig. 2c ; F 8,24 =26.8, ANOVA. P =0.038, Tukey–Kramer HSD) and cluster formation by unicells, which declined in frequency by 97%. Together, these observations demonstrate that experimentally evolved C. reinhardtii possess a novel multicellular life cycle consisting of alternating phases: a dispersal phase, in which clusters reproduce via motile unicellular propagules and do not grow larger and a growth phase, during which clusters produce few propagules and instead increase in cell number ( Fig. 3a ). 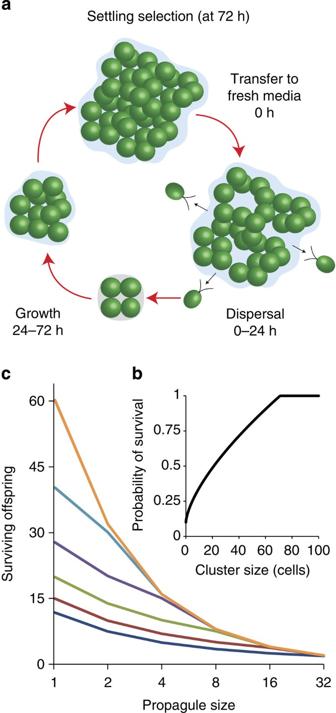Figure 3: Life cycle evolution. (a) Life cycle of multicellularC. reinhardtii.Shortly after settling selection and transfer to fresh medium, motile unicells disperse away from the parent cluster. These cells lose motility and develop into clusters prior to the next round of settling. (b) Our model predicts that smaller clusters should experience reduced survival, up to a cluster size of ~70 cells (survival is assured for larger clusters). (c) Shown are the number of surviving offspring a single 64-cell cluster is calculated to produce as a function of propagule size and the number of doublings propagules undergo prior to settling selection (dark blue: 1, red: 2, green: 3, purple: 4, light blue: 5, orange: 6). Despite the reduced survival of smaller clusters during settling selection, unicellular propagules maximize the number of surviving offspring a cluster can produce. Figure 3: Life cycle evolution. ( a ) Life cycle of multicellular C. reinhardtii. Shortly after settling selection and transfer to fresh medium, motile unicells disperse away from the parent cluster. These cells lose motility and develop into clusters prior to the next round of settling. ( b ) Our model predicts that smaller clusters should experience reduced survival, up to a cluster size of ~70 cells (survival is assured for larger clusters). ( c ) Shown are the number of surviving offspring a single 64-cell cluster is calculated to produce as a function of propagule size and the number of doublings propagules undergo prior to settling selection (dark blue: 1, red: 2, green: 3, purple: 4, light blue: 5, orange: 6). Despite the reduced survival of smaller clusters during settling selection, unicellular propagules maximize the number of surviving offspring a cluster can produce. Full size image Cultures of C. reinhardtii are known to form nonmotile ‘palmelloid’ colonies under some environmental conditions [26] , but these palmelloids differ in two important ways from the multicellular clusters observed in this experiment. First, palmelloids in wild-type C. reinhardtii form plastically in response to conditions such as predator presence [27] , organic acids [28] , Ca 2+ deficiency, chelating agents and high phosphate concentrations [29] . Our multicellular clusters form obligately in culture conditions in which wild-type C. reinhardtii form no such clusters. Clearly, the difference between our cluster-forming strain and the single-celled strains of the control populations are genetic, not plastic. Second, the morphology of our multicellular clusters is distinct from that of palmelloids. Palmelloids typically consist of 4–16 cells [28] and are thought to result from the failure of a single generation of daughter cells to break out of the mother cell wall [26] . Our multicellular clusters, in contrast, can contain >100 cells (mean of 58 cells at 72 h; Fig. 2c ), include multiple mitotic generations of descendants of the founding cell ( Fig. 1e ) and are not held together by a parental cell wall but rather by a gelatinous extracellular matrix (individual cells are still encapsulated by their own cell walls; Fig. 1b ). Life history model To determine whether unicellular propagules confer a fitness benefit in the absence of genetic conflict, we examined the direct effect of propagule size on reproductive success. Multicellular C. reinhardtii face a classic resource allocation trade-off: more offspring can be produced if fewer cells are invested in each propagule [15] , but under conditions in which large size is favored (for example, settling selection or predation [23] ), smaller size may diminish offspring survivorship. For multicellular C. reinhardtii , larger cluster size increases survival during settling selection for clusters up to ~70 cells, at which point their settling speed is sufficient to guarantee survival ( Fig. 3b ). We mathematically determined the propagule size that maximizes the number of surviving offspring a 64-cell cluster can produce in our selection regimen ( sensu Lack, 1947 (ref. 30 )). We modelled 64-celled clusters because they are similar in size to our evolved strain at 72 h (mean of 58 cells; Fig. 2c ), but are more mathematically tractable. We varied the amount of growth propagules obtained prior to selection from 1–6 doublings, because greater growth should reduce the cost of smaller propagule size. Despite their lower relative survival, we find that unicellular propagules still maximize the number of surviving offspring a cluster can produce under all resource conditions modelled ( Fig. 3c ), and are especially beneficial when growth prior to settling selection is substantial. This direct benefit favors the production of unicellular propagules, even in the absence of within-cluster genetic conflict. Once a single-cell bottleneck has evolved, genetic variation will be efficiently segregated between multicellular individuals. This limits the potential for subsequent genetic conflict to arise, facilitating the evolution of traits normally susceptible to social exploitation (for example, cellular division of labour). A unicellular bottleneck may therefore arise as an early life history adaptation to maximize direct reproductive success, creating lineages that are preadapted to the resolution of intercellular conflicts as a side-effect. Using experimental evolution, we find that simple algal multicellularity can arise in as little as 219 days in a species that has never had a multicellular ancestor. Multicellular C. reinhardtii display a novel two-stage life cycle in which motile unicellular propagules disperse shortly after transfer to fresh medium, then undergo successive rounds of mitosis to form nonmotile, multicellular clusters bound by an extracellular matrix. The multicellular life cycle that evolved in our system bears some similarity to one of the most distant relatives of Volvox within the colonial volvocine algae. The four cells in a Basichlamys sacculiferum cluster are held together by a gelatinous matrix produced by the mother cell [31] but dissociate into single cells before forming new clusters [32] . Attachment of cells through the production of such an extracellular matrix has been predicted to be one of the first steps in volvocine evolution [10] , [33] . If this change preceded the evolution of genetic control of cell number, it is possible that the ancestors of the volvocine algae were similar to our evolved C. reinhardtii . Despite strong selection, substantial evolutionary responses to selection occurred in just 1 of 10 populations under settling selection within 219 days ( Fig. 1a ). Surprisingly, unique major adaptive responses to selection are not uncommon in experimental evolution [34] , [35] , [36] , [37] and the topic of idiosyncratic responses to selection remains a major topic of investigation [8] , [38] , [39] . An excellent example is the evolution of citrate catabolism in E. coli (a highly beneficial trait) in 1 out of 12 experimental populations after 31,500 generations of evolution in citrate-containing medium [40] . No citrate utilization occurred in the other 11 populations, even after 8,000 further generations of selection. Even though E. coli was unlikely to evolve the ability to use citrate, this selection experiment clearly shows that the possibility existed. These results are not surprising for traits that require multiple specific mutations, thereby engendering historical contingency for adaptation [41] . In our Chlamydomonas experiment, we observe the evolution of a multicellular lineage that has a greatly increased rate of settling, consistent with the selection regime. As in the study by Blount et al . [40] , we observe a singular evolutionary outcome that demonstrates an evolutionary possibility. Specifically, we observe that simple multicellularity can evolve rapidly in an organism that has never had a multicellular ancestor, and that a single-cell bottleneck can evolve without selection to minimize among-cell genetic conflict. Even though multicellularity has evolved dozens of times in the last 3.5 billion years, this transition is still rare (occurring, most recently, ~200 MYA in the brown [5] and the volvocine [6] algae). Although it is possible that a control population could evolve multicellularity in a few months, this would be an unexpected outcome given that hundreds of independent lineages in the genus Chlamydomonas (including C. reinhardtii ) have failed to do so over hundreds of millions of years. More broadly, our finding that simple multicellularity can evolve in less than a year in both Chlamydomonas and Saccharomyces [24] suggests that genetic barriers (for example, few mutational paths to multicellularity) may be less restrictive than ecological barriers, namely a lack of persistent selective advantages for cellular clusters. Unicellular bottlenecks are present in distantly related multicellular lineages [11] , [12] , [13] , and appear to be a critical step in the evolution of multicellular complexity. The unicellular bottleneck limits genetic diversity, and hence genetic conflict, among the cells of extant multicellular organisms [1] , [11] , [12] , [17] , [18] , [20] , [21] , [42] , and ensures that all cells constituting a multicellular individual share a common developmental history and environment. Both of these factors facilitate the transition to multicellular-level selection and the subsequent evolution of multicellular complexity. Little, however, is known about the origin of the single-cell bottleneck in extant taxa. Here we demonstrate that a unicellular bottleneck can evolve during the first stage of this major evolutionary transition, and that it is adaptive even in the absence of genetic conflict, maximizing the reproductive success of the nascent multicellular individual. Given the unicellular ancestry of all multicellular organisms, this trait may evolve especially rapidly if the single-celled stage can be co-opted from the ancestral unicellular form (such as motile unicells; Fig. 1c,d ). In combination with recent work demonstrating the origin of multicellular clusters capable of Darwinian evolution [24] , [43] , our findings suggest that multicellular complexity may evolve more readily than previously thought. Generating an outbred unicellular population We generated an outbred population of Chlamydomonas reinhardtii to start with a high level of standing genetic variation. Genetically diverse wild-type Chlamydomonas strains were obtained from the Chlamydomonas Resource Center at the University of Minnesota. We performed all pair-wise crosses between mating type (+) strains CC-2932, CC-2936, CC-2937, CC-125, CC-1690, CC-2343, CC-2344, CC-4414 and mating type (–) strains CC-2938, CC-2931, CC-2935, CC-124, CC-1691, CC-2290, CC-2342 following standard procedures [26] . With the exception of the following, all crosses were successful: CC-2343 × CC-2931, CC-2343 × CC-2938, CC-2343 × CC-1691, CC-2343 × CC-2290, CC-4414 × CC-2935, CC-4414 × CC-2342, CC-2937 × CC-2938. Successful F1 crosses were inoculated into 25 ml of TAP medium [26] in a 125 ml flask and grown for 4 days under lights at 22.5 °C with shaking at 150 r.p.m. This population was put through one round of sexual reproduction (within-population mating), and the resulting outbred F2 population was used as the starting point for the selection experiment. Selection protocol Twenty replicate populations were established in a 24-well plate of TAP medium (2 ml per well). Cultures were grown under lights at 22.5 °C for 72 h without shaking. The four extra wells were filled with 2 ml of uninoculated TAP medium. To limit edge effects, replicate populations were rotated through the plate, moving one well to the right every transfer. Cultures from wells on the right-hand edge were inoculated into the left-most well one row down. After 72 h of growth, cultures were homogenized by pipetting (1 ml aspiration, three times per well), 1 ml was then removed and placed in a sterile 1.5-ml microcentrifuge tube. This was centrifuged at 100 g for 5 s, then the upper 900 μl was removed by pipette and discarded. The remaining 100 μl was then inoculated into 1.9 ml TAP medium and grown for 72 h without shaking. All populations were put through one round of sexual reproduction (within-population mating) at transfer 15, but due to inconsistent recovery from sporulation, this step was not repeated during the remainder of the experiment. Time-lapse microscopy All microscopy was performed on an Olympus IX70 inverted microscope with a SPOT Flex 64 MP camera. Clusters were inoculated into an eight-well Nunc Lab-Tek II chamber slide containing 0.5 ml fresh TAP media at a low density (1:100 dilution). Images were acquired either every 30 s ( Fig. 1e ) or every second ( Supplementary Movie 1 ) for at least 16 h. Quantifying cluster movement Time-lapse images were opened in ImageJ as a virtual stack, then thresholded to separate cell biomass from background. Using the Calculator Plus plugin, we subtracted the image at time ( t +1 s) from time t and then measured the non-overlapping area. Non-moving cells were removed by subtraction. The difference between images (in μm 2 ) is a measure of the distance that the cluster moved in the last second. By dividing by the maximum measured value, we generated an index of relative movement (ranging from 0, no movement, to 1). Measuring cluster size At transfer 73, 10 single-strain isolates were randomly isolated from the population containing multicellular Chlamydomonas (no isolates were unicellular). Single-strain isolates were purified through three rounds of single-colony isolation on TAP agar plates. Each isolate was inoculated into 2 ml TAP medium from storage on an agar slant and grown for 72 h to create a master stock that would be used for subsequent inoculations. Master stocks were refrigerated at 4 °C for 24 h prior to their first use. Three replicate populations were generated by inoculating 100 μl of each master stock into 2 ml of fresh TAP media, staggering each inoculation by 24 h. All populations were grown for 3 days and then transferred to fresh TAP with settling selection (as described above). These Chlamydomonas were then grown for 0, 24, 48 or 72 h and harvested simultaneously, then imaged microscopically. Cluster size was determined by diluting Chlamydomonas fivefold into fresh TAP medium and imaging two non-overlapping fields of view at × 4 magnification. All microscopy was performed in a hemocytometer to avoid flattening clusters. Cluster volume was determined by calculating the volume of best-fit ellipses (following the procedure of Ratcliff et al . [44] ). Cluster volume was expressed in units of cell volumes ( Fig. 2c ) by dividing cluster volume by the volume of a single cell (315 μm 3 ), which was determined by measuring the size of 1,938 motile unicells (see below). Mean cluster size for one isolate was an outlier (8.5-fold larger than the average of the other nine isolates at t 0 , caused by the inclusion of a large cluster at this time point). This outlier isolate was removed from the analysis. Determining the frequency of motile unicells The frequency of motile unicells was determined in a manner similar to cluster size. Chlamydomonas were cultured in the same manner (use of master stocks to start replicate populations), but inoculation timing was not staggered. Instead, replicate populations were destructively harvested after 0, 2, 4, 6, 8, 24, 48 and 72 h of growth. All populations were loaded onto a hemocytometer and 1–2 fields of view imaged at × 4 magnification. Cluster size was determined using best-fit ellipses. Two images separated by 0.2 s were acquired, and the former image subtracted from the latter using the Calculator Plus plugin in ImageJ, removing any cells that did not move. Motile unicells were then counted and their volume determined using ImageJ. The fraction of the population that were motile unicells was determined by dividing the volume of all motile unicells in the sample by the total volume of Chlamydomonas in the sample. Sequencing five unlinked loci in 10 isolates We sequenced the following regions to estimate the number of lineages represented in the 10 multicellular isolates (locus names from the C. reinhardtii genome database on phytozome.net ): ~370 bp of cell wall protein pherophorin-C1 (locus Cre17.g717900) including the 5′ untranslated region (UTR), ~350 bp of pherophorin-C3 (g6305; chromosome 6) including the 5′ UTR, ~380 bp of pherophorin-C4 (Cre12.g549000) including the 5′ UTR, ~810 bp of pherophorin-C5 (Cre05.g238650) including the 5′UTR, and ~810 bp of the beta subunit of ATP synthase (chloroplast). We extracted genomic DNA using the DNEasy Plant Maxi Kit (Qiagen) and PCR-amplified the regions of interest using DreamTaq 2 × master mix (Thermo Scientific) with the primers in Table 1 . PCR cycles included an initial denaturation of 2 min. at 95 °C followed by 36 cycles of 30 s denaturation at 95 °C, 30 s primer annealing at 45–54 °C and 2 min extension at 72°C, and a final extension of 10 min at 72 °C. PCR products were purified using the PCRExtract Mini Kit (5Prime Inc., Gaithersburg, MD, USA) and Sanger sequenced using the PCR primers at the University of Washington High Throughput Sequencing Center. Across the five unlinked loci we sequenced, the sequences of all 10 isolates were identical, suggesting that selection had reduced the initially heterogeneous population to a single lineage by the end of the experiment. Modeling the effect of propagule size on recruitment Probability of cluster survival: cluster survival during settling selection depends on being in the lower 100 μl of the 1 ml volume undergoing centrifugation. There are two ways that this can occur: first, clusters can settle through their growth medium into this lower fraction. Second, they start out there prior to settling selection. We can measure the probability that a cluster’s settling distance will result in survival (getting to the lower 100 μl) quite simply: assuming that the starting location within the medium column is random, then the expected survival rate is the distance travelled by the cluster as a fraction of the total distance to safety. The distance a cluster travels can be calculated as tv c , where t is the duration of settling (in seconds) and v c is the speed of the cluster. Assuming that a cluster can be approximated by a sphere, we use Stokes’ law to calculate v c as: where v c is the settling rate of the cluster (in cm s −1 ), g is gravitational acceleration (in cm s −2 ), μ is the dynamic viscosity of water (in g cm s −1 ), ρ d and ρ m are the average density of the cluster and growth media (in g cm −1 ), respectively and d is the cluster diameter (in cm). For this calculation we used g =98,100, d ranged from 0.00085 (diameter of a single cell, determined from the size of 1,938 motile unicells, see Methods) to 0.01, ρ d =1.05 (density measurement of Chlamydomonas from ref. 45 ), ρ m =1 and μ=0.01. The probability a cluster will settle far enough to survive selection can be written as: where t is the duration of settling (in seconds) and h is the maximum distance a cluster will have to travel to survive settling selection (in cm). This is the long-run expectation that a cluster starting out in a random position in the water column will travel far enough to reach the transfer fraction (lower 100 μl). In our experiments, t= 5 and h= 1.85. The fraction of clusters surviving settling selection simply by being in the volume transferred to fresh media prior to selection ( γ ) can be calculated as the transfer volume divided by the total selection volume. In our experiment, 10% of the selection volume was transferred. The probability that a cluster of size n will survive settling ( p s,n ) is the sum of the probabilities of settling far enough to survive, and starting out already in the transferred volume: Offspring recruitment: Offspring recruitment (number of progeny surviving settling selection) was determined for a 64-cell cluster. We assumed that during the reproductive phase of the life cycle, all cells in the cluster dispersed in propagules of size 1, 2, 4, 8, 16 or 32 cells. These then underwent 1–6 doublings ( δ ) before settling selection (the high end of this range corresponds to the amount of growth seen in just 24 h, see Fig. 1e ). Propagule size at settling selection ( n ) can be determined by multiplying the initial size of the propagule ( s p ) by the fold-increase in size prior to selection: ( s p 2 δ ). Offspring recruitment ( R ) is then the number of propagules produced by a cluster, modified by their probability of surviving settling selection given their size: where s c is cluster size prior to propagule dispersal. Of course, these results depend on the agent selecting for large size. For example, if phagotrophic predators strongly prefer unicellular prey, then a single-celled bottleneck may not be optimal. Accession codes: The DNA sequences have been deposited in GenBank nucleotide database under the accession codes KF767355 – KF767404 sequences. How to cite this article: Ratcliff, W.C. et al . Experimental evolution of an alternating uni- and multicellular life cycle in Chlamydomonas reinhardtii . Nat. Commun. 4:2742 doi: 10.1038/ncomms3742 (2013).